Anisotropic structure of the order parameter in FeSe0.45Te0.55revealed by angle-resolved specific heat The central issues for understanding iron (Fe)-based superconductors are the symmetry and structure of the superconducting gap. So far the experimental data and theoretical models have been highly controversial. Some experiments favor two or more constant or nearly constant gaps, others indicate strong anisotropy and yet others suggest gap zeros ('nodes'). A unique method for addressing this issue, and one of very few methods that are bulk and angle resolved, is measuring the electronic-specific heat in a rotating magnetic field. In this study, we present the first such measurement for an Fe-based high- T c superconductor. We observed a fourfold oscillation of the specific heat as a function of the in-plane magnetic field direction. Our results are consistent with the expectations for an extended s-wave model, with a significant gap anisotropy on the electron pockets and the gap minima along the ΓM (Fe–Fe bond) direction. The discovery of high-temperature superconductivity in iron (Fe) pnictides [1] was arguably the most important event in the physics of superconductivity since the discovery of cuprate superconductors. Despite impressive progress in the last 2 years, the most basic question: what are the symmetry and structure of the order parameter?—remains unanswered. Yet, without firmly answering this question further theoretical advance, most importantly, identification of the pairing mechanism, becomes essentially impossible. We already have some clues on these issues (see papers by Mazin et al . [2] , Kuroki et al . [3] , Wang et al . [4] and Mazin [5] for detailed discussions). Indeed, it seems highly unlikely that very similar materials with the same main structural element, the FeAs or FeSe planes, would have qualitatively different pairing symmetries (quantitative differences are of course possible). For several Fe-based high- T c superconductor (FeBSC), the nuclear magnetic resonance data have positively identified the parity of the superconducting state as singlet, essentially leaving only two possibilities for the angular momentum of the Cooper pairs: L=0 (s-wave) and L=2 (d-wave). These two, in turn, can divide into several different subtypes. Specifically, in the tetragonal symmetry several symmetry distinguishable versions of the d-wave pairing are allowed, with the basis functions transforming as x 2 − y 2 , xy , and xz , yz or xz ± yz ( xz ± iyz is excluded by the μSR experiments, which would have detected a spontaneous magnetization below T c in a chiral state). Furthermore, substantial indirect evidence has been accumulated against the relevant d-wave symmetries. First, the Josephson current is finite and sizeable along the z -direction in some of the FeBSCs [6] . This excludes any order parameter that integrates to zero over x and y at every given z . Second, angular resolved photoemission spectroscopy shows that in many FeBSC the gap is fairly isotropic on each Fermi surface (FS) pocket [7] , [8] . This, again, excludes x 2 − y 2 and xy near the surface, and, by implication, in the bulk. Preliminary data exist also for a 11 material similar in composition to ours, although these data are still incomplete with regard to the electron-like FS [9] . Third, absence of the Wohlleben (paramagnetic Meissner effect) in some 1111 materials indicates that weak links in polycrystalline samples have predominantly 0 phase shifts, whereas both x 2 − y 2 and xy symmetries imply roughly 50:50 distributions of 0 and π phase shifts [10] . At the same time, multiple evidences indicate the existence of unpaired quasiparticles (QPs) at small energies, sometimes all the way down to nearly zero energies [11] , [12] . The most natural explanation would be that the excitation gap has nodes somewhere on the FS, and the nodal areas provide low-energy QPs. Yet another explanation, which is now popular, is that the low-energy excitation are due to the pair-breaking effects of defects and impurities in the scenario of s ± pairing [13] . Arguably, the most sensitive probe of the low-energy excitation structure, thermal conductivity and penetration depth measurements seems to point to nodal or nearly nodal states in three FeBSCs, KFe 2 As 2 [14] , LaFePO [15] , [16] and BaFe 2 (As,P) 2 [17] , and to full gaps with various degrees of anisotropy in many others [18] , [19] , [20] , [21] . It has been suggested, based on the anisotropy of the penetration depth, that some materials may have an accidental nearly horizontal nodal line within an extended s-wave model [22] . At this point, it becomes truly indispensable to address the angular structure of the order parameter directly, and in the bulk. Indeed, as explained below, in this way one can distinguish between an isotropic gap or a horizontal nodal line, on the one hand, and a vertical nodal line, on the other. If other experiments (e.g., thermal conductivity) suggest the presence of nodes, and there is no ab plane angular dependence, this indicates a horizontal nodal line. If, however, an angular dependence is detected, this demonstrates the presence of vertical nodes, and pinpoints their location on the FS. If, finally, such a dependence is present, but angle-integrated experiments exclude nodes, one concludes that the material has a highly anisotropic nodeless order parameter (with known location of gap minima). This is invaluable information, but how can it be harvested? On the theory side, most attempts to deduce the angular structure of the order parameter from model calculations on 1111 and 122 materials roughly agree that deep minima or gap nodes may appear in some parameter range (see paper by Chubukov and Eremin [23] and references therein), usually along the ΓM direction on the outer electron FS. Chubukov and Eremin [23] have pointed out that if the order parameter can be expanded in spherical harmonics around the M point, then in the lowest order, the gap minima can only occur along the ΓM direction, either on the outer or on the inner surface. The most effective and accurate techniques for addressing the angular structure of the order parameter rely on probing thermodynamic properties in a rotating in-plane magnetic field. A review on the angle-dependent thermal conductivity in unconventional superconductors can be found in the study by Matsuda [24] . Recently, Matsuda et al . [25] have measured the thermal conductivity in such a field in BaFe 2 (As 1−x P x ) 2 . They concluded that gap nodes exist on the electronic FS, centered around the M point. In this paper we have used a different approach, angle-resolved specific heat (ARSH) measurements, and we have selected a material for which thermal conductivity at low temperature indicates an anisotropic order parameter without nodes [26] , FeSe x Te 1− x . We find a strong fourfold anisotropy in ARSH. Given the thermal conductivity data [26] , we conclude that FeSe x Te 1− x has a strongly anisotropic s-wave nodeless gap, with deep (deeper than ~50% of the maximal gap) minima along the ΓM (the Fe–Fe bond in the real space) directions. Furthermore, using the fact that tunneling data [27] indicate a full gap of ~1.4 meV with no detectable subgap density of states (DOS) in the same compound, we suggest that the minima are more likely to occur on the inner electron FS. Samples and characterization The FeSe 0.45 Te 0.55 single crystals were grown using the self-flux method. Details regarding the growth of the samples are given in the Methods section. 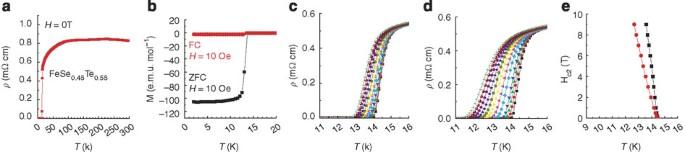Figure 1: Sample characterizations. (a) The temperature dependence of resistivity in a wide temperature region for the FeSe0.45Te0.55sample. It shows a sharp resistive transition atTc,mid≈ 14.5 K. (b) Zero-field-cooling (ZFC) and field-cooling (FC) magnetization measured in the field of 10 Oe. The magnetization in the low-temperature region is flat and the Meissner screening volume is almost 100%. (c,d) Resistivity in magnetic fields (c) H||ab and (d) H||c. The curves from the right to left correspond to magnetic fields of 0, 0.2, 0.5, and from 1 to 9 T with increments of 1 T. The random error bars of resistivity and magnetization are ±0.0005 mΩ cm and ±0.0008 e.m.u. mol−1, respectively. (e) The upper critical fields Hc2(T) for in-plane and out-of-plane field orientations, with error bars of ±0.05 T. The black line shows H||ab, whereas the red line refers to H||c. In Figure 1a , we plot the resistivity in a wide temperature range; a broad bump appears in the intermediate temperature regime, which seems to be an intrinsic feature of the FeSe x Te 1− x system and has been reported by others [28] . The resistive transition at 14.5 K is narrower than 0.5 K (10–90% ρ n ). The magnetization measured in zero-field-cooling process demonstrates a perfect Meissner effect, as shown in Figure 1b . The magnetic field dependence of the resistivity is shown in Figure 1c (H||ab) and Figure 1d (H||c). The broadening of the resistive transition is quite small, indicating a high upper critical field. In the Figure 1e, we show the temperature dependence of the upper critical fields with two field orientations. In H||c, the superconducting transition temperature decreases by ~1.79 K at 9 T, but only by 0.91 K in H||ab. The slope of the upper critical field is d H c2, ab ( T )/d T | T = T c =−10.4 T/K, and d H c2,c ( T )/d T | T = T c =−5.26 T/K, yielding an anisotropy ~2. 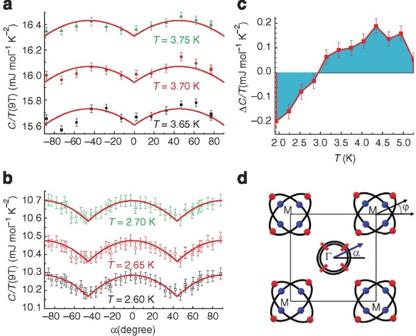Figure 2: Angle dependence of specific heat coefficient and proposed positions of gap minimum. Data measured at (a) 3.65, 3.7 and 3.75 K and (b) 2.6, 2.65 and 2.7 K in the in-plane magnetic field of 9 T, whereαis the angle between the field and the Fe-Se-Fe bond direction. Fourfold oscillations are observed and the amplitude is ~0.12 mJ mol−1K−2(T=2.6 K). The fourfold oscillations were repeatable in two separate samples. The maximum ofC/Tis located at about zero degrees (H||Fe-Se-Fe), whereas the sign of the oscillations is reversed when the temperature is increased to 3.7 K. The red lines are theoretical simulations (seeSupplementary Methods) using thed(x2−y2) order parameter Δk=Δ0(coskx−cosky). The actual functional dependence is not important: any reasonable model that yields the gap nodes located at the same directions46,47would produce a very similar angular dependence. (c) The temperature dependence of the difference ofC/Tat 0° and 45°, a crossover is clearly seen at ~2.9 K. The random error bars (after the averaging of 300 data points) of specific heat are ±0.04 mJ mol−1K−2. (d) Possible locations of nodes or gap minima suggested by our data are shown by the red and blue balls on the folded electron Fermi pockets, and by red segments on the hole Fermi surfaces. The ellipticity of the electron pockets is exaggerated in this drawing. The sharp magnetic and resistive transitions, together with the very small residual-specific heat coefficient γ 0 (see Methods ), demonstrate the good quality of the sample and allow us to proceed with the ARSH measurements, as shown in Figure 2a–c . Figure 1: Sample characterizations. ( a ) The temperature dependence of resistivity in a wide temperature region for the FeSe 0.45 Te 0.55 sample. It shows a sharp resistive transition at T c,mid ≈ 14.5 K. ( b ) Zero-field-cooling (ZFC) and field-cooling (FC) magnetization measured in the field of 10 Oe. The magnetization in the low-temperature region is flat and the Meissner screening volume is almost 100%. ( c , d ) Resistivity in magnetic fields ( c ) H||ab and ( d ) H||c. The curves from the right to left correspond to magnetic fields of 0, 0.2, 0.5, and from 1 to 9 T with increments of 1 T. The random error bars of resistivity and magnetization are ±0.0005 mΩ cm and ±0.0008 e.m.u. mol −1 , respectively. ( e ) The upper critical fields H c2 (T) for in-plane and out-of-plane field orientations, with error bars of ±0.05 T. The black line shows H||ab, whereas the red line refers to H||c. Full size image Figure 2: Angle dependence of specific heat coefficient and proposed positions of gap minimum. Data measured at ( a ) 3.65, 3.7 and 3.75 K and ( b ) 2.6, 2.65 and 2.7 K in the in-plane magnetic field of 9 T, where α is the angle between the field and the Fe-Se-Fe bond direction. Fourfold oscillations are observed and the amplitude is ~0.12 mJ mol −1 K −2 ( T =2.6 K). The fourfold oscillations were repeatable in two separate samples. The maximum of C / T is located at about zero degrees (H||Fe-Se-Fe), whereas the sign of the oscillations is reversed when the temperature is increased to 3.7 K. The red lines are theoretical simulations (see Supplementary Methods ) using the d ( x 2 − y 2 ) order parameter Δ k =Δ 0 (cos k x −cos k y ). The actual functional dependence is not important: any reasonable model that yields the gap nodes located at the same directions [46] , [47] would produce a very similar angular dependence. ( c ) The temperature dependence of the difference of C/T at 0° and 45°, a crossover is clearly seen at ~2.9 K. The random error bars (after the averaging of 300 data points) of specific heat are ±0.04 mJ mol −1 K −2 . ( d ) Possible locations of nodes or gap minima suggested by our data are shown by the red and blue balls on the folded electron Fermi pockets, and by red segments on the hole Fermi surfaces. The ellipticity of the electron pockets is exaggerated in this drawing. Full size image Theory of ARSH In a type-II superconductor, applying a magnetic field (shown by an arrow in Fig. 2d ) induces vortices extending along the field direction, with a supercurrent flowing in the perpendicular plane. Due to the motion of this flowing electron condensate, the local QP DOS, N ( ϵ ), in the area surrounding the vortex core will be affected by a Doppler shift with the energy δE = m v s · v F , as N ( ϵ )= N ( ϵ 0 ± δE ), with δE for band number ( i ) given by [29] , [30] , [31] Here α characterizes the direction of the external field, ω is the winding angle of the supercurrent around the vortex, and is the normalized (to the average value of the Fermi velocity in the corresponding band), x - ( y -) component of the Fermi velocity. The Doppler shift energy scale is defined as [31] , where Φ 0 is the flux quantum, and a is a geometrical factor taking 0.465 for the triangle vortex lattice; ρ is a dimensionless variable characterizing the distance from the vortex core. This energy shift, as discussed for instance by Graser et al . [32] , leads to the energy shift of the DOS curve, and thus, for a clean BCS superconductor, to the following equation for the DOS at the Fermi level (in units of the normal DOS): where the first averaging is performed over the unit cell of the vortex lattice and the second over the FS. For a nodal or quasi-nodal superconductor, the main k dependence comes from the order parameter in the denominator; therefore, we have kept this subscript explicitly in Δ. The maximal value of ρ is (ref. 32 ) 1; therefore, in principle, in a nodal superconductor, there will always be directions near the nodes, where N (0) is non-zero (where ), reaching its normal value precisely at the nodal points. An important thing to appreciate is that there is always some residual DOS at the nodes, which is simply enhanced by the effect of the magnetic field, and the net effect of this enhancement is strongest when all nodes are 'excited', and not just a few of them. This leads to the slightly counterintuitive result that N (0) is maximal when the magnetic field is aligned with an antinodal (and not a nodal) line. This result holds only for sufficiently low temperatures and fields. For a given magnetic field, there is a reversal temperature, T *, and at higher temperatures N (0) is maximal when the magnetic field is aligned with nodal lines. This result appears to be quite universal: it was obtained in the Doppler shift approximation [33] , [34] , as well as in more accurate approaches [35] , [36] , [37] . The exact value of T *, however, is rather model sensitive and the only way to determine in which regime one actually works is to repeat the measurements at different temperatures and until the actual reversal has been obtained. This has been performed, for instance, in the study by An et al . [38] for CeCoIn 5 , and we also have found a reversal as a function of temperature in our experiment. This allowed us to pinpoint the positions of the gap minima with complete certainty. As opposed to the position of the minima, the detailed gap structure is much harder to determine; it is important to remember that even in the most favorable cases disorder or three-dimensional dispersion considerably reduce the amplitude of the oscillations compared with the original calculated value for a two-dimensional d-wave gap (10% is usually considered to be a reasonable upper limit for realistic systems) [32] , [33] , [34] . In fact, the ARSH has been successfully applied in identifying the nodal gap structure in such superconductors as CeRhIn 5 [39] and YNi 2 B 2 C [40] (in both cases about 5% oscillations have been detected). Note that in a 'quasinodal' case, where the gap does not have true nodes, but has a very small value along particular directions, the above discussion still holds, as long as . Measurements of ARSH In Figure 2a–c, we present our experimental results. We rotate the sample with the FeSe plane parallel to the direction of a fixed magnetic field and measure the variation of the specific heat. As shown in Figure 2a,b , the specific heat coefficient γ = C / T shows clear fourfold oscillations as a function of the in-plane 9 T magnetic field. At low temperatures, T =2.6–2.7 K, minima appear when the field is along the ΓM direction, but when the temperature is increased to about 3.65–3.75 K, oscillations are reversed, with the maxima along the ΓM directions (see Fig. 2a ). This is extremely important, because recent theoretical estimates [23] , [41] have placed the reversal temperature, T * , at a rather low temperature, whereas our data unambiguously prove that 2.7 K< T *<3.6 K. In order to show this, in Figure 2c , we present the difference of C / T between the data collected at α =0° and 45°. One can see a clear crossover between the two regions at about 2.9 K in H =9 T. Because of this, we can say with complete certainty that the gap minima are located along the ΓM lines. As an additional test, we have measured the specific heat of the same sample in H =0, as well as in an isotropic superconductor Nb in H =0.4 T while rotating the sample. Within the error bars, we have not seen any oscillations of ARSH in either case. Therefore, we believe that the oscillations shown in Figure 2 really reflect the gap structure in FeSe 0.45 Te 0.55 . As discussed above, the observation of the oscillations of specific heat tells us that the minimum gap should be smaller than the Doppler shift energy, E H . Our local density approximation calculations yield an average Fermi velocity that is similar for the two hole sheets and the outer electron sheet, varying between 2.5×10 5 and 2.6×10 5 m s −1 , and for the inner electron sheet. Assuming a many-body renormalization of the order of 2–3, and H =9 T, we estimate E H to be between 1 and 2 meV. Thus, these results present direct bulk evidence of a strong gap anisotropy with nodes or deep minima. Now, we consider the FS topology in this system. Calculations [42] and angular resolved photoemission spectroscopy [9] indicate the same generic Fermiology as in Fe pnictides, which includes two sets of the FSs: the hole one contains two or three roughly cylindrical pockets around the Γ point at the center of the Brillouin zone (0,0), and the electron one consists of two overlapping warped elliptical cylinders near the M point (π,π). 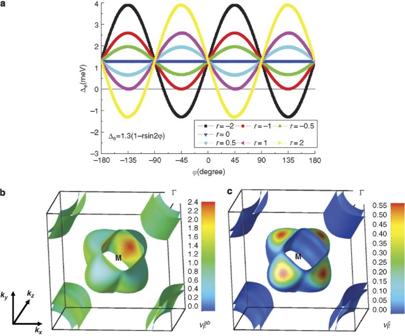Figure 3: Fermi surface (FS) and the variation of the order parameter. (a) The angle dependence of the gap on the electron pocket around M(π,π), based on the extendeds-wave gap function Δe(ϕ)=Δ0[1−rsin 2ϕ] with Δ0=1.3 meV. The minima are located at 45° (Fe–Fe or ΓM direction), if 1>r>0. For the negativer, maxima are located at −45°. For |r|>1, instead of minima, sign-changing nodes appear. (b,c) The FSs of FeSexTe1−x, as calculated from first principles. Note the strong warping of the outer electron pocket (now shown in the center of the picture for a better view). The shading represents the function, which controls the electronic transport in the ab-plane (b), and the same for(caxis transport) (c). The angular dependence of gap on the electron pocket around this point is shown in Figure 3a . The points near which the gap nodes can be located, according to our ARSH data, are shown by the colored markers in Figure 2d . Note that the ellipticity in FeSe x Te 1− x is rather small compared, say, to 122 materials, so the effects of the anisotropy in the FS and the Fermi velocity should be very weak (the calculated FSs are shown in Fig. 3b,c ; in the diagrammatic representation of Fig. 2d, the ellipticity is intentionally exaggerated). Therefore, we conclude that the oscillations of the specific heat in our samples are not due to an anisotropic Fermi velocity [35] , [36] . This is corroborated by the fact that the fourfold oscillations of the specific heat reverse their sign when the temperature is changed slightly. The anisotropy of the Fermi velocity cannot change appreciably between 2.6 and 3.7 K. Figure 3: Fermi surface (FS) and the variation of the order parameter. ( a ) The angle dependence of the gap on the electron pocket around M(π,π), based on the extended s -wave gap function Δ e ( ϕ )=Δ 0 [1− r sin 2 ϕ ] with Δ 0 =1.3 meV. The minima are located at 45° (Fe–Fe or ΓM direction), if 1> r >0. For the negative r , maxima are located at −45°. For | r |>1, instead of minima, sign-changing nodes appear. ( b , c ) The FSs of FeSe x Te 1− x , as calculated from first principles. Note the strong warping of the outer electron pocket (now shown in the center of the picture for a better view). The shading represents the function , which controls the electronic transport in the ab-plane ( b ), and the same for ( c axis transport) ( c ). Full size image A canonical x 2 − y 2 ( xy in the one-Fe unit cell) d-wave pairing on the hole-FS would readily explain our data (shown by the red lines in Fig. 2a,b ). Indeed, it would have created the nodal lines at the right spots in both hole bands, and electron pockets (red and blue balls, and red dashes in Fig. 2d ). However, as discussed in the introduction, there is convincing evidence against this pairing state. Another viable alternative is that the nodal lines form on the electron FSs, as indicated also by recent Raman scattering measurements [43] , [44] , at the points marked by the red and blue balls on the electron pockets ( Fig. 2d ). Indeed, a number of model calculations [45] , [46] , [47] predict nodes at the electron FS in some parameter range. The gap structure in these calculations is set by the orbital composition of the electron bands in the unfolded Brillouin zone, and nodes appear roughly where the character changes from the xy /( x 2 − y 2 ) orbitals to the xz / yz orbitals. In Figure 2a,b we compare simulated curves with the nodes located at the ΓM line, α=45° (e.g., d-wave) with experiment (see the Supplementary Methods for the description of simulations). We observe that this scenario is consistent with the experiment, as is an extended s -wave model with the nodes located within ±5° from 45° (not shown here). However, nodes that are farther away from α =45° do not describe the data well enough. On the other hand, existing calculations [47] suggest that for the parameters appropriate for FeSe no nodes are present at all. Thermal conductivity [26] indicates that there are no zero nodes in Fe(Se,Te) superconductors, but deep minima. All in all, this points to a scenario with no nodes, but deep minima on either inner or outer electron barrels, or both, as shown by the blue or red balls in Figure 2d . Assuming that the order parameter varies smoothly with the angle, one can expand it as a function of winding angle on the relevant FS [23] , [41] . If, as suggested by model calculations, the anisotropic part is in the gap on the electron pockets, we can expand it as [23] , Δ e ( ϕ )=Δ 0 [1− r sin 2 ϕ ], where the winding angle ϕ is counted with respect to the Fe-Se-Fe direction, as shown in Figure 2d , and r controls the gap anisotropy. In Figure 3a, we show the angle dependence of the gap on the electron pocket centered at M(π,π), taking Δ 0 =1.3 meV. For | r |<1, there are no nodes, but minima at ϕ =±45°, located on the outer ( r >0) or inner ( r <0) barrels. For | r |>1, pairs of nodes appear on both sides of these directions and they are moving away as the anisotropy parameter r grows. We should note several points here: (1) model calculations for 122 compounds suggest r >1 (refs 46 , 47 ); (2) a model calculation for FeSe suggests 0< r <1 (in fact, r ~0.6) [47] (3) thermal conductivity suggests no nodes, that is [26] , | r |<1 and (4) scanning tunneling microscope (STM) suggests an isotropic gap ( r ~0) [27] . It is worth noting that from the point of view of our experiment we cannot distinguish the sign of r : nodes or minima on the inner barrel or on the outer barrel would produce practically the same ARSH spectra. Finally, as the oscillations can only be observed when the Doppler shift energy is larger than or comparable with the minimum value of the gap, the gap minima should be ~1 meV or less. Using the gap value estimated from STM, 1.4 meV, we find that | r |>0.25. In principle, our data are consistent with the functional renormalization group calculations given in the study by Wang et al . [47] (and it is reasonable to assume that random phase approximation calculations would give similar results), as well as with thermal conductivity measurements, suggesting that r is large, but not larger than 1. However, STM experiments bring in a new dimension as they do not detect any subgap DOS at all. Interestingly, it is possible to reconcile all experimental results among themselves (but not with the model calculations), if we assume that r is large but negative, and take into account the fact that the STM current is dominated by those parts of the FS that have sizeable Fermi velocity along the tunneling direction (crystallographic c axis). As Figure 3c shows, the Fermi velocity along c axis is non-negligible for the outer barrel only, whereas for the inner barrel (and for both hole FSs, for that matter), it is vanishingly small. Thus, if the minima are on the inner barrel, they would not be seen in the STM experiment, but would be in ours, and, interestingly, in the thermal conductivity experiment: as Figure 3b shows, if the inner barrel does not completely dominate the in-plane transport, it makes the largest contribution to it. An alternative explanation would be that the minima exist only in the bulk (but not near the surface as detected by the STM measurements), and live on the outer barrels, as predicted by theory, but disappear near the surface. To summarize, we have measured the angle-resolved low-temperature-specific heat in an external in-plane magnetic field. We find that, as the field direction rotates with respect to the crystallographic axes, fourfold oscillations of the specific heat appear, indicating a strong fourfold anisotropy of the order parameter in FeSe 0.45 Te 0.55 . The results can be formally interpreted in terms of a nodal d xy gap at the Γ-FS, but such interpretation is not consistent with other experiments on the same compound. A consistent interpretation can be provided in terms of an order parameter that has deep minima (deeper than roughly 50% of the maximal gap) on the electronic FSs, located at the crossing point of the ΓM direction (the Fe–Fe bond direction) in the Brillouin zone and the electron pockets. We cannot distinguish between the two possibilities, that the minima are located on the outer electron barrels or on the inner ones. The former one is consistent with existing model calculations, whereas the latter is consistent with the STM tunneling data on the same compound, and with thermal conductivity. Sample growing The FeSe 0.45 Te 0.55 single crystals were grown by self-flux method. Powders of Fe, Se and Te were mixed in stoichiometric ratio and filled in a ceramic crucible. The weighing, mixing and pressing procedures were performed in a glove box filled with highly pure Ar gas, in which both O 2 and H 2 O concentrations were <0.1 p.p.m. The crucible with the starting materials was sealed in an evacuated quartz tube. It was heated up to 720 °C, kept for 10 h, and further heated up to 1,050 °C for melting the material, then it was slowly cooled down to 720 °C at a rate of 5 °C h −1 before the furnace was shut off. The samples used for the present measurements were 2.6 mm×4.7 mm×0.35 mm (thickness) in dimension. Well-cleaved crystals were sealed in an evacuated quartz tubes again and annealed at 400 °C for more than 300 h. All annealed samples show sharp superconducting transitions, as shown by the diamagnetic measurements. Measurements and verifications The specific heat was measured using the relaxation technique based on a home-made measuring puck, which rotates with the sample in the dewar of a Quantum Design instrument PPMS-9T. Due to a careful design, during the rotation, the FeSe planes of the sample are always parallel to the magnetic field. The measurement puck was tested by measuring Nb. The results were fully consistent with those reported in the literature. During the measurements for each angle, the sample was cooled down in a magnetic field, with the angle between the crystallographic axis and the direction of the magnetic field fixed. After the measurement had been finished, the sample was warmed up for changing the magnetic field (all measurements were performed in the field-cooling mode) and rotated to another angle. In order to suppress the noise, the measurements were repeated 300 times for each data point shown in Figure 2a,b . In order to check that the observation of the fourfold oscillations in the magnetic field in FeSe 0.45 Te 0.55 was not an artifact, we measured the specific heat at H =0 by rotating the sample FeSe 0.4 Te 0.60 , and a conventional superconductor, Nb, in an in-plane field H =0.4 T. As shown in Supplementary Figure S2 , the data from Nb at H =0.4 T do not present any discernable oscillations. The same happens for the sample FeSe 0.4 Te 0.60 at H =0 and T =2.6 K (data not shown here). Our analysis of different contributions to the specific heat of the FeSe 0.45 Te 0.55 is illustrated in Supplementary Figure S3 , where we present the specific heat coefficient γ = C / T measured at H =0 and 9 T (H||ab) in wide temperature region, as well as Supplementary Table S1 . It is clear that the specific heat anomaly at about 12 K (middle point of the specific heat anomaly) is rather sharp. The low-temperature data at H =0 T has a slight upturn, which is given by the Schottky anomaly (the entropy contributed by the paramagnetic centers with s =1/2). Although a linear extrapolation of the data in the high-temperature region can give a reasonable assessment of all terms, we shall still do the global fitting for the data measured at H =0. The total specific heat C total includes the residual term γ 0 T , the phonon part C ph / T = βT 2 , the Schottky anomaly part γ Sch . The specific heat resulting from the superconducting part is assumed to be negligible in this low-temperature region. Therefore, we have where g is the g -factor, taking two for the case s =1/2 and assuming weak spin-orbital coupling, H eff is the effective crystal field, n is a prefactor related to the number of paramagnetic centers. Using the above equation, we get a good fit to the data at H =0, yielding γ 0 =1.66 mJ mol −1 K −2 , β =0.924 mJ mol −1 K −4 , n =21 mJ mol −1 K −2 , H eff =3.1 T. As shown in the inset of Supplementary Figure S3 , after removing the Schottky anomaly, the data exhibit roughly linear behavior, extrapolating to γ 0 at T =0 K. No upturn in H =9 T is observed, indicating that the Schottky anomaly is weak. Based on above equation, the Schottky term in our experiment at H =9 T is much smaller than that in H =0 T in the temperature region of 2.6–2.7 K, in which we collected the ARSH data. Even if the Schottky anomaly is present, it should not give rise to any particular angular dependence. How to cite this article: Zeng, B. et al . Anisotropic structure of the order parameter in FeSe 0.45 Te 0.55 revealed by angle-resolved specific heat. Nat. Commun. 1:112 doi: 10.1038/ncomms1115 (2010).